Microtubule and cortical forces determine platelet size during vascular platelet production Megakaryocytes release large preplatelet intermediates into the sinusoidal blood vessels. Preplatelets convert into barbell-shaped proplatelets in vitro to undergo repeated abscissions that yield circulating platelets. These observations predict the presence of circular-preplatelets and barbell-proplatelets in blood, and two fundamental questions in platelet biology are what are the forces that determine barbell-proplatelet formation, and how is the final platelet size established. Here we provide insights into the terminal mechanisms of platelet production. We quantify circular-preplatelets and barbell-proplatelets in human blood in high-resolution fluorescence images, using a laser scanning cytometry assay. We demonstrate that force constraints resulting from cortical microtubule band diameter and thickness determine barbell-proplatelet formation. Finally, we provide a mathematical model for the preplatelet to barbell conversion. We conclude that platelet size is limited by microtubule bundling, elastic bending, and actin-myosin-spectrin cortex forces. Human adults have ∼ 1 trillion circulating blood platelets (PLTs), and, because the lifespan of an individual PLT is only 8–10 days, 100 billion new PLTs are produced daily from bone marrow megakaryocytes (MKs) to maintain their 150–400×10 9 l −1 counts in whole blood. PLTs are anucleate discoid cells 1.5–3 μm in diameter. Among their primary functions, PLTs serve as the 'band-aids' of the bloodstream and respond to blood vessel injury by changing shape, secreting their granule contents, and aggregating to form a PLT clot. These responses, while advantageous for haemostasis, can become undesirable, if they cause tissue ischemia or infarction. Despite a growing list of PLT-associated disorders, resulting from higher-than-normal or lower-than-normal PLT counts [1] , the terminal stages of PLT production and ultimate determinants of PLT size remain unknown. The current model of PLT formation recognizes that, on reaching maturity, bone marrow MKs will extend, through junctions in the lining of blood sinuses, long, branching proPLTs. These dynamic intermediate structures are consisted of tandem arrays of slender tubular projections cored by microtubule bundles with PLT-sized swellings at their ends. ProPLT-producing MKs in culture release intermediate barbell structures that yield individual PLTs [2] , [3] . ProPLTs have been identified extending and releasing into blood vessel sinusoids both in vitro and in vivo [4] , [5] , and are therefore believed to mature in the circulation [3] , [6] . We have recently identified a new intermediate stage called the prePLT in the maturation process. PrePLTs are anucleate discs 3–10 μm across that reversibly convert into barbell-shaped proPLTs to divide and form two PLTs [7] . Here we show that circular-prePLTs and barbell-proPLTs are present in human whole blood, and quantify them using a laser scanning cytometry assay. We propose and test a biological model for terminal PLT production that predicts marginal microtubule coil diameter and thickness determine barbell-proPLT formation and regulate PLT size. Lastly, we provide a mathematical and computational model that is based on the balance of microtubule bundling forces, elastic bending forces, and actin-spectrin-myosin cortex forces to describe the mechanism of circular-prePLT to barbell-proPLT conversion. Identification of the critical prePLT size To establish the morphometric characteristics of circular-prePLTs and barbell-proPLTs that will be used to quantify them in whole blood, we employed a quantitative immunofluoresence microscopy-based assay. Released proPLT cultures were isolated as previously described [7] , spun down onto poly- L -lysine-coated glass coverslides, and probed for the MK lineage-specific β1-tubulin isoform to delineate the cell periphery. Five-by-five composite images were generated from individual images taken at ×20 magnification and collected for at least 3 different samples ( Fig. 1a ). Individual cells were thresholded based on a binary image mask and analysed across multiple morphometric parameters including area, circularity, perimeter and number. 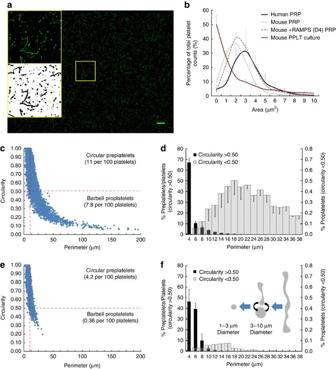Figure 1: Quantitative immunofluorescence microscopy of mouse and human proPLTs. (a) Composite image of mouse FLC proPLTs. Objects were identified by their fluorescence intensity, and thresholded on a binary mask to quantify area, circularity, perimeter, and number. (b) Validation of approach using mouse/human PLT controls. (c) Circularity/perimeter measurements from mouse FLC cultures. (d) A minimum perimeter for barbell-proPLTs and maximum diameter for circular-prePLTs of∼10 μm was used to establish a∼3-μm diameter threshold to distinguish circular-prePLTs from PLTs in mouse FLC cultures. (e) Human PRP reveal PLT-intermediates in whole blood. (f) Human PRP. Analyses were performed for at least three independent samples. Error bars represent 1s.d. about the mean. Scale bar, 50 μm. Figure 1: Quantitative immunofluorescence microscopy of mouse and human proPLTs. ( a ) Composite image of mouse FLC proPLTs. Objects were identified by their fluorescence intensity, and thresholded on a binary mask to quantify area, circularity, perimeter, and number. ( b ) Validation of approach using mouse/human PLT controls. ( c ) Circularity/perimeter measurements from mouse FLC cultures. ( d ) A minimum perimeter for barbell-proPLTs and maximum diameter for circular-prePLTs of ∼ 10 μm was used to establish a ∼ 3-μm diameter threshold to distinguish circular-prePLTs from PLTs in mouse FLC cultures. ( e ) Human PRP reveal PLT-intermediates in whole blood. ( f ) Human PRP. Analyses were performed for at least three independent samples. Error bars represent 1s.d. about the mean. Scale bar, 50 μm. Full size image Quantitative immunofluoresence microscopy of released proPLT cultures was validated using human and mouse PLT controls ( Fig. 1b ). To distinguish intermediates in PLT production, objects identified by quantitative immunofluoresence microscopy in murine proPLT cultures were categorized as resting PLTs, circular-prePLTs, or barbell-proPLTs based on their circularity and perimeter measurements ( Fig. 1c ). Precise measurements of mouse proPLT culture intermediates revealed a minimum perimeter for barbell-proPLTs of ∼ 10 μm ( Fig. 1d ), which translates to a circular diameter of ∼ 3 μm. This size limit, below which barbell-proPLTs are rarely detected, was defined as the critical prePLT size, and represents the tipping point for competing forces that govern twisting of the resting PLT's marginal microtubule coil about its midsection to form the barbell-proPLT structure. An ∼ 3-μm diameter threshold was therefore established to distinguish discoid PLTs, which are incapable of undergoing barbell-proPLT conversion, from their circular-prePLT progenitors. Examination of human PLT-rich plasma (PRP) using this approach predicted the presence of circular-prePLTs and barbell-proPLTs in whole blood ( Fig. 1e ), which adhered to the size constraints governing circular-prePLT to barbell-proPLT conversion established in murine cell cultures ( Fig. 1f ). Large PLTs often occur concomitantly with periods of PLT depletion in humans [8] and various forms of MK processes, and proPLTs are present in cytospin preparations of human PRP [9] . Nevertheless, because barbell-proPLTs are not detected in human blood smears, it is unclear whether these circulate in blood, and their role in thrombocytopenia has not been studied. To demonstrate the existence of circular-prePLTs and barbell-proPLTs in the circulation, and establish the experimental conditions for their detection and subsequent quantification, whole blood from the same human donor was collected into 10% AJ buffer or sodium citrate, EDTA, and heparin tubes (anticoagulant) ( n =3). Representative Giemsa-stained blood smears in Fig. 2a demonstrate the presence of barbell-proPLTs and circular-prePLTs in AJ buffer and sodium citrate, but not in EDTA- and heparin-treated blood. EDTA has been shown to affect proPLT concentration in the venous and arterial circulation of rats and cause PLT sphering [10] . Immunofluorescence microscopy images of β1-tubulin-stained PRP from EDTA- and Heparin-treated blood confirmed this, and revealed smaller PLTs with thicker/brighter microtubule coils ( Fig. 2b ). These results account for why barbell-proPLTs have not previously been reported in human blood smears and establish important experimental preconditions for quantification of PLT production intermediates from whole blood. 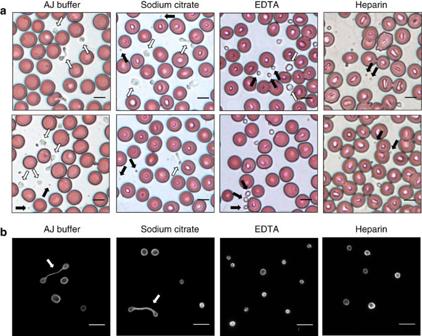Figure 2: Giemsa-stained blood smears from anticoagulant-treated human whole blood. (a) PLT intermediates were present in AJ buffer and sodium citrate, and absent in EDTA and heparin anticoagulant-treated blood smears. EDTA-treated PLTs are sphericized. (b) Immunofluoresence images of β1-tubulin-stained PRP. EDTA-treated PLTs were smaller, with more constricted microtubule coils. PLTs are indicated by black arrows, whereas circular-prePLTs or barbell-proPLTs are indicated by white arrows. Scale bar, 5 um. Figure 2: Giemsa-stained blood smears from anticoagulant-treated human whole blood. ( a ) PLT intermediates were present in AJ buffer and sodium citrate, and absent in EDTA and heparin anticoagulant-treated blood smears. EDTA-treated PLTs are sphericized. ( b ) Immunofluoresence images of β1-tubulin-stained PRP. EDTA-treated PLTs were smaller, with more constricted microtubule coils. PLTs are indicated by black arrows, whereas circular-prePLTs or barbell-proPLTs are indicated by white arrows. Scale bar, 5 um. Full size image Quantification of PLT intermediates in blood To overcome the quantification limitations of immunofluorescence microscopy, and more accurately identify specific intermediate forms in PLT production from whole blood, we developed a laser scanning cytometry assay. Human PRP was isolated and probed for β1-tubulin on poly- L -lysine-coated glass coverslides. Supplementary Fig. S1a illustrates the laser scanning cytometry analysis work flow for the detection and quantification of intermediates in PLT production from PRP. Resting PLTs, circular-prePLTs, and barbell-proPLTs were differentially gated based on morphological and signal-level dependent scattergram analysis from which a representative image gallery was generated ( Fig. 3a ). Barbell-proPLTs in human whole blood were distinguished from circular/discoid objects based on their unique barbell morphology, and ranged in perimeter from roughly 10–32 μm (or 3–10 μm in diameter if assumed to convert into circular objects). These observations support previous measurements of barbell-proPLTs and circular-prePLTs in cell culture presented in Fig. 1 . Circular-prePLTs in human whole blood were therefore distinguished from discoid PLTs based on their ability to convert into barbell shapes [7] , and gated based on the empirically determined diameter of ∼ 3 μm. This enabled us to determine circular-prePLT and barbell-proPLT counts in whole blood, which comprised 3.63 and 0.05% of PLT counts, respectively ( Fig. 3b ). 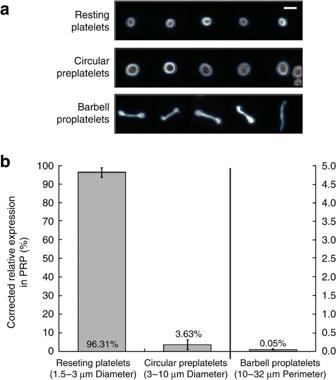Figure 3: Quantification of PLT intermediates in human venous blood. (a) Image gallery of resting PLTs, circular-prePLTs, and barbell-proPLTs differentially gated based on morphological and signal-level dependent scattergram analysis. (b) Resting PLT, circular-prePLT and barbell-proPLT counts from human PRP normalized for total object counts. Analyses were performed for at least three independent samples. Error bars represent 1 s.d. about the mean. Scale bar 3 μm. Figure 3: Quantification of PLT intermediates in human venous blood. ( a ) Image gallery of resting PLTs, circular-prePLTs, and barbell-proPLTs differentially gated based on morphological and signal-level dependent scattergram analysis. ( b ) Resting PLT, circular-prePLT and barbell-proPLT counts from human PRP normalized for total object counts. Analyses were performed for at least three independent samples. Error bars represent 1 s.d. about the mean. Scale bar 3 μm. Full size image Biological model of proPLT conversion The demonstration that prePLTs can undergo barbell-proPLT conversion while PLTs cannot, led us to propose the following biological model of vascular PLT production: Force constraints resulting from cortical MT band diameter and thickness determine barbell formation and account for circulating discoid PLT size. This model makes three fundamental biological predictions regarding the mechanism of proPLT conversion. If peripheral microtubule coil thickness is kept constant, large PLTs will undergo barbell-proPLT conversion whereas small PLTs will not. Thinner peripheral microtubule coils will be more able to overcome resistance to elastic bending forces that limit barbell-proPLT conversion than thicker microtubule coils. The elongating microtubule bundle is deformed by the external compressive pressure of the actin-myosin-spectrin cortex. ProPLT elongation by bone marrow MKs, and circular-prePLT to barbell-proPLT conversion are primarily driven by reorganization of the microtubule cytoskeleton. The development of an in vitro assay to separate circulating human PLT intermediates from red blood cells (RBCs) ( Supplementary Methods ) enabled us to finely assess vascular proPLT/prePLT ultrastructure by thin section and negative stain electron microscopy. Whole blood-derived prePLT/proPLTs were cytoplasmically indistinguishable from mature PLTs and large PLT-like intermediates from mouse MK cell cultures ( Fig. 4a,b ) and contained comparable numbers of peripheral microtubules ( Fig. 4c,d ; Supplementary Fig. S2 ). PLTs from Filamin A knock-out (KO) mice were included as a positive control because they are known to be larger than normal circulating mouse PLTs and contain thicker microtubule coils [11] . These data establish the experimental preconditions by which to test biological prediction 1. 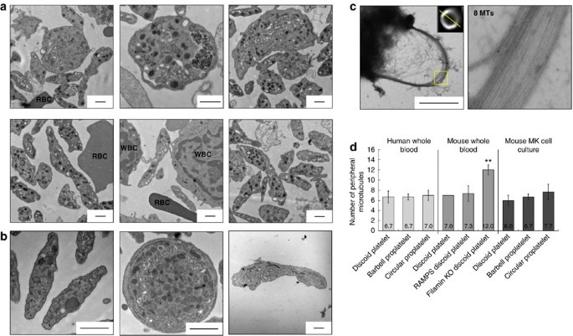Figure 4: Ultrastructural analysis of PLT intermediates. (a) Thin-section EMs of human whole-blood PLTs, circular-prePLTs (top), and barbell-proPLTs (bottom). (b) EMs of mouse blood PLTs (left), FLC circular-prePLT (middle) and FLC barbell-proPLT (right). (c) Negative-stained EM and immunofluorescence micrograph with linescan (insert) of human whole-blood PLT used to measure the number, size and fluorescence intensity of the peripheral microtubule band. (d) Quantification of negative-stained EMs revealed 6–8 peripheral microtubules in PLTs, barbell-proPLTs and circular-prePLTs. PLTs from Filamin A KO mice shown as a positive control. Analyses were performed for at least three independent samples. Error bars represent one standard deviation about the mean. Statistical significance was established using a one-tailed Student'st-test for paired samples (**P<0.01). Scale bar, 1 μm. Figure 4: Ultrastructural analysis of PLT intermediates. ( a ) Thin-section EMs of human whole-blood PLTs, circular-prePLTs (top), and barbell-proPLTs (bottom). ( b ) EMs of mouse blood PLTs (left), FLC circular-prePLT (middle) and FLC barbell-proPLT (right). ( c ) Negative-stained EM and immunofluorescence micrograph with linescan (insert) of human whole-blood PLT used to measure the number, size and fluorescence intensity of the peripheral microtubule band. ( d ) Quantification of negative-stained EMs revealed 6–8 peripheral microtubules in PLTs, barbell-proPLTs and circular-prePLTs. PLTs from Filamin A KO mice shown as a positive control. Analyses were performed for at least three independent samples. Error bars represent one standard deviation about the mean. Statistical significance was established using a one-tailed Student's t -test for paired samples (** P <0.01). Scale bar, 1 μm. Full size image Biological prediction 1 stipulates that above a threshold diameter elongating microtubules in the PLT marginal band are capable of overcoming bending energies needed to undergo barbell-proPLT conversion, whereas, below this threshold diameter, PLTs remain discoid. To increase PLT diameter, human/murine PRP was cultured at 37 °C with gentle rotation in a humidified incubator for 0 and 6 h [12] , and analysed by LSC. 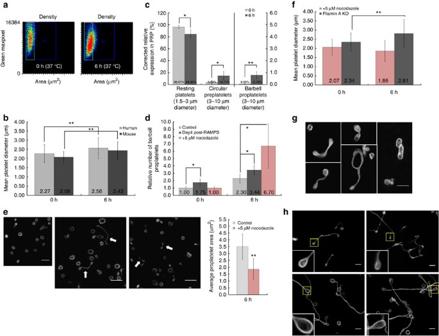Figure 5: Structural determinants of proPLT conversion. (a) Density scattergrams of human PRP. PLTs and circular-prePLTs are represented by a cyan and blue box, respectively. (b) Mean diameter of resting PLTs increased following incubation at 37 °C. (c) Increasing PLT size resulted in lower relative PLT counts, higher circular-prePLT counts and increased barbell-proPLT conversion in human PRP at 37 °C. (d) Mouse PRP at 37 °C. Larger PLTs from RAMPS-treated mice produced more barbell-proPLTs than WT controls. (e) Relative to DMSO 0 h. (left) and 6 h. (middle) controls, 5 μM nocodazole treatment (right) generated increased numbers of smaller barbell-proPLTs (white arrows). (f) Mean diameter of nocodazole-treated and filamin KO mouse PLTs following incubation at 37 °C. (g) PRP from filamin A KO mice demonstrate larger, irregular shaped proPLTs at concentrations∼40% of WT controls. (h) Relative to DMSO control (top-left), actin-stabilizing drug jasplankinolide (top-right), and destablizing drugs latrunculin (bottom-left) and cytochalasin D (bottom-right) decreased/increased proPLT end size, respectively. Analyses were performed for at least three independent samples. Error bars represent 1 s.d. about the mean. Statistical significance was established using a one-tailed Student'st-test for paired samples (*P<0.05, **P<0.01). Scale bar, 5 μm. Figure 5a shows a representative density scattergram of these cultures over time, and confirms microtubule coil enlargement at 37 versus 22 °C control ( Supplementary Fig. S3a ). Increased mean PLT diameter (μm) for human and mouse PRP cultures are illustrated in Fig. 5b and explains lower-resting PLT and increased circular-prePLT counts, described in Fig. 5c . Increasing microtubule coil diameter resulted in more barbell-proPLT conversion relative to 22 °C controls ( Supplementary Fig. S3b ), and supports our biological prediction. Samples were normalized for total object counts to address differences in PLT numbers between human replicates. These observations agree with earlier findings by Schwertz et al . [12] , and may partly account for why increases in PLT size and barbell-proPLT number have not previously been reported in the literature for PLT units, which are typically stored at 22 °C. Figure 5: Structural determinants of proPLT conversion. ( a ) Density scattergrams of human PRP. PLTs and circular-prePLTs are represented by a cyan and blue box, respectively. ( b ) Mean diameter of resting PLTs increased following incubation at 37 °C. ( c ) Increasing PLT size resulted in lower relative PLT counts, higher circular-prePLT counts and increased barbell-proPLT conversion in human PRP at 37 °C. ( d ) Mouse PRP at 37 °C. Larger PLTs from RAMPS-treated mice produced more barbell-proPLTs than WT controls. ( e ) Relative to DMSO 0 h. (left) and 6 h. (middle) controls, 5 μM nocodazole treatment (right) generated increased numbers of smaller barbell-proPLTs (white arrows). ( f ) Mean diameter of nocodazole-treated and filamin KO mouse PLTs following incubation at 37 °C. ( g ) PRP from filamin A KO mice demonstrate larger, irregular shaped proPLTs at concentrations ∼ 40% of WT controls. ( h ) Relative to DMSO control (top-left), actin-stabilizing drug jasplankinolide (top-right), and destablizing drugs latrunculin (bottom-left) and cytochalasin D (bottom-right) decreased/increased proPLT end size, respectively. Analyses were performed for at least three independent samples. Error bars represent 1 s.d. about the mean. Statistical significance was established using a one-tailed Student's t -test for paired samples (* P <0.05, ** P <0.01). Scale bar, 5 μm. Full size image As mice exhibit a greater proportion of large, young PLTs in their circulation that may be equivalent to prePLTs following antibody-induced thrombocytopenia versus untreated controls ( Fig. 1b ) [13] , we hypothesized that these should form a greater number of barbell-proPLTs in circulation and in culture. To test this hypothesis PRP was isolated from mouse whole blood 4 days before and following rabbit anti-mouse platelet serum (RAMPS) infusion, and stored at 37 °C for 0 and 6 h. Expectedly, a significantly larger number of barbell-proPLTs were present in RAMPS-treated mice versus untreated controls, both at 0 and 6 h post-collection ( Fig. 5d ). Representative immunofluoresence microscopy images of β1-tubulin-stained PRP from these samples are outlined in Supplementary Fig. S3c . Restricting microtubule coil enlargement, by comparison, should result in fewer barbell-proPLTs in culture. To test this hypothesis human whole blood was collected directly into sodium citrate, EDTA, and heparin tubes, and either stored in the same tube for 6 h at 37 °C or transferred into a new anticoagulant-treated tube every hour to restrict PLT enlargement. Representative immunofluoresence microscopy images of β1-tubulin-stained PRP from these samples are outlined in Supplementary Fig. S3d . Hourly treatment of human whole blood with EDTA or heparin blood was shown to keep PLTs at a smaller size, and inhibited barbell-proPLTs relative to the sodium citrate control. These results support our biological prediction, and demonstrate that force constraints resulting from cortical microtubule band diameter regulate barbell-proPLT formation. If barbell-proPLT formation is determined by the balance of microtubule bundling and elastic bending forces, thinner peripheral microtubule coils will more easily undergo barbell-proPLT conversion than thicker ones. To inhibit microtubule polymerization, PLTs were incubated with increasing concentrations of nocodazole, and cultured at 37 °C for 6 h. Nocodazole-treated PLTs did not become larger ( Fig. 5f ), and resulted in increased numbers of smaller barbell-proPLTs relative to the DMSO control ( Fig. 5d and e ), which agree with our predictions. Alternatively, we looked at filamin A KO mouse PLTs, which are significantly larger than their wild-type (WT) controls ( Fig. 5f ) [11] , contain thicker microtubule coils ( Fig. 4d ), and were shown to increase proportionately in size, following incubation at 37 °C for 6 h ( Fig. 5f ). Barbell-proPLTs in these samples were present at a concentration of ∼ 40% that of WT controls, were larger, and formed irregular shapes in culture ( Fig. 5g ). These results demonstrate that microtubule bundling forces and elastic bending forces determine critical prePLT size. For peripheral microtubule coil lengthening to buckle, driving proPLT formation, the expansion force that is generated by microtubule coil sliding and/or polymerization must be checked by an equally strong compressive force deriving from the cell cortex. To test this prediction, proPLTs were treated with the actin-destabilizing drugs latrunculin and cytochalasin D for 2 h, which were shown to increase proPLT end size, and the actin-stabilizing drug jasplankinolide, which was shown to decrease proPLT end size, relative to the DMSO control ( Fig. 5h ). We have also recently shown that barbell proPLTs treated with the spectrin disrupting peptide spα2N1 are unable to retain their barbell shape and collapse into a circular prePLT form [14] . These observations confirm that elongating microtubule bundles in the peripheral coil are being deformed by the external compressive pressure of the actin-myosin-spectrin cortex during proPLT conversion. Mathematical model of proPLT conversion As barbell-proPLT conversion is regulated by microtubule coil diameter and thickness, we hypothesized that the balance between the elastic bending forces of the peripheral microtubule bundle and the effective actin-spectrin-myosin cortex tension determine barbell-proPLT shape and critical prePLT size ( Fig. 6a ). To test this hypothesis, we developed a mathematical model of circular-prePLT deformation during which the perimeter of the peripheral microtubule bundle was increased while cell area was maintained constant by a rigid actin-myosin-spectrin cortex ( Fig. 6b ; Supplementary Movie 1 ). As the microtubule bundle elongated, the middle part of the cell narrowed, until the opposite parts of the microtubule bundle touched, forming a barbell-proPLT structure. On reaching this point, microtubule associated proteins crosslink the microtubule bundle creating a 'corridor' between the lobes of the barbell-shaped cell. In vivo , the peripheral microtubule coil twists about its midsection to form the barbell-proPLT structure [7] . To validate that our model was accurately representing this, the energy of a twisted microtubule bundle of two microtubules as a function of the helical pitch was modelled, and the energy minimum it described corresponded to the predicted pitch of the twisted microtubule bundle ( Supplementary Fig. S4 ). These results demonstrate that twisting of the microtubule bundle in the barbell-proPLT shaft can lower the sum of the bundling elastic energies to account for this process in vivo . 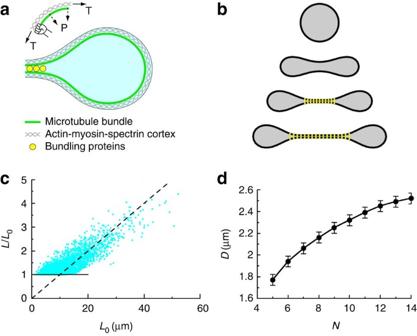Figure 6: Mathematical modelling of barbell-proPLT conversion. (a) Schematic of force balance as outlined by Laplace's Law (P=pressure,T=cortex tension). (b) Simulated shapes in proPLT conversion. After corridor formation, microtubule-bundling proteins (short yellow lines) 'zip up' the corridor. From top to bottom, the ratio of shown cell perimeter to initial, circular, perimeter:L/L0=1, 1.5, 2, 2.5. (c) Circularity relation.L0=perimeter of the initial circular-prePLT,L=perimeter of the barbell-proPLT. Solid line:L/L0=1. Dashed line:L/L0=L0/(10 μm). (d) Simulated PLT diameter vs number of microtubules in the bundle. Analyses were performed for at least three independent samples. Error bars represent 1 s.d. about the mean. Figure 6: Mathematical modelling of barbell-proPLT conversion. ( a ) Schematic of force balance as outlined by Laplace's Law ( P =pressure, T =cortex tension). ( b ) Simulated shapes in proPLT conversion. After corridor formation, microtubule-bundling proteins (short yellow lines) 'zip up' the corridor. From top to bottom, the ratio of shown cell perimeter to initial, circular, perimeter: L / L 0 =1, 1.5, 2, 2.5. ( c ) Circularity relation. L 0 =perimeter of the initial circular-prePLT, L =perimeter of the barbell-proPLT. Solid line: L / L 0 =1. Dashed line: L / L 0 = L 0 /(10 μm). ( d ) Simulated PLT diameter vs number of microtubules in the bundle. Analyses were performed for at least three independent samples. Error bars represent 1 s.d. about the mean. Full size image This computational model makes a number of biological predictions that are supported by our data ( Supplementary Methods ). First, calculations show that the effective force needed to expand and bend the peripheral microtubule bundle during circular prePLT to barbell-proPLT conversion is inversely proportional to prePLT area: f ∝ L 0 −2 ( Supplementary Fig. S4 ). Assuming that this force is generated by microtubule motors (for example, cytoplasmic dynein) and microtubule polymerization, and does not scale with circular-prePLT size (or changes relatively slowly with the size), our model predicts that, below a certain size threshold, this force will be insufficient to elongate the microtubule bundle. In other words, while microtubule number and diameter regulate PLT size, pre-PLT intermediates are not required to have thicker peripheral microtubules. Increasing the number of peripheral microtubules, however, will result in terminal platelets of a larger proportional size owing to their inability to undergo further barbell-proplatelet conversion. Indeed, Figs 1d and 6c confirm this hypothesis for our proPLT cultures and indicate that the respective critical prePLT diameter in these samples is ∼ 10 μm. This is not an absolute threshold, and critical prePLT size is predicted to depend on the number of microtubule motors and peripheral microtubules in the cell. Second, these data indicate that when circular-prePLT size is greater than critical, the perimeter of the resulting proPLT scales as L ∝ L 0 −2 ( Fig. 6c ). This model lets us explain this scaling in one of three ways: total amount of tubulin scales with prePLT area; proPLTs stop deforming when the motor force density that scales as f mot ∝ L 0 −1 (constant number of motors distributed over distance L ) decreases to the necessary microtubule tensile force f ∝ L 0 −2 cell area remains constant throughout PLT morphogenesis. Third, final PLT size can be explained by this model as resulting from the balance between the bundling force and microtubule elastic bending force. When characteristic protein forces and microtubule rigidity are factored in, the predicted PLT radius is calculated to be in the micron range, as observed. Fourth, this model predicts that PLT size increases slowly as the microtubule number in the peripheral bundle cross-section grows. This agrees with measurements of WT and filamin A KO PLTs that show, when the microtubule number increases from 7 to 12 ( Fig. 4d ), baseline PLT size increases from 2.08 ( Fig. 5b ) to 2.34 μm ( Fig. 5f ). During cell culture at 37 °C, PLT diameters are increased, possibly driven by microtubule sliding and/or polymerization, resulting in barbell-proPLT formation. Figure 6d summarizes this relationship by illustrating computed PLT size as a function of microtubule number. This model establishes the mechanism describing a terminal stage in PLT production and makes important predictions that can be tested to account for well-defined differences in mean PLT size among different mouse strains, and compared with mouse/human macrothrombocytopaenias to identify important cytoskeletal interactions affecting normal PLT production. We present here three new insights into the terminal mechanisms of PLT production. First, we accurately quantify circular-prePLTs and barbell-proPLTs in human blood from high-resolution fluorescence images by a laser scanning cytometry assay. This advance overcomes the quantification limitations of microscopy and qualitative limitations of flow cytometry that have previously been employed, and shifts the paradigm of PLT release from bone marrow MKs towards large PLT-like intermediates in the blood. From it, we conclude that circular-prePLTs are dynamic intermediate structures in platelet production. Given the relatively low concentration of barbell-proPLTs in venous blood, it is possible that, once circular-prePLTs convert into barbell-proPLTs, abscission is rapid. Alternatively, prePLTs may become trapped in the micro-capillaries of the bone marrow, lung and/or spleen where intravascular shear forces can drive PLT production. Indeed, reports of higher PLT counts in post-pulmonary vessels suggests that the lung may be a milieu for terminal PLT formation [15] . Second, we show that twisting microtubule-based forces driving circular-prePLT to barbell-proPLT conversion are governed by two major biophysical properties: microtubule coil diameter and microtubule coil thickness. Indeed, large PLTs from patients with Gray PLT syndrome, May-Hegglin anomaly, and Epstein's syndrome contain 10–20-fold increased numbers of peripheral microtubule coils relative to normal human PLTs, which agree with our predictions [16] . Many giant PLTs also contain peripheral microtubules, organized like balls of yarn, that may explain why the majority of these cells have a spherical rather than discoid form [16] . Last, these observations have allowed us to address what forces determine barbell-proPLT formation and establish a mechanism for how the final PLT size is established. Barbell-proPLT conversion is an elaborate and complex process that defines the morphology and ultrastructure of circulating PLTs. PLT number and size are often inversely proportional, and others have shown that the PLT cytoskeleton can regulate PLT size and numbers through specific transmembrane receptor interactions. GPIb, for example, is complexed to the actin-binding protein filamin A and is known to have an important role in maintaining the normal cytoskeletal architecture of resting PLTs [17] , [18] . In Bernard Soulier Syndrome genetic abnormalities of the GPIb-IX-V complex, particularly the GPIbα subunit that contains the Von Willebrand factor and thrombin-binding sites, results in fewer and larger PLTs [1] . As normal numbers of MKs are generally found in the bone marrow of these patients, it is likely that the macrothrombocytopaenia is related to an error in the terminal stages of PLT production. Moreover, the novel identification of an autosomal dominant macrothrombocytopaenia associated with PLT dysfunction in Glanzmann's Thrombasthaenia [19] raises interesting questions about the role of GPIIIa and its beta terminal domain in proPLT formation and PLT release. Myosin IIA, the non-muscle myosin heavy chain product of the MYH9 gene, has also been implicated in restraining proPLT formation in developing MKs [20] . In the case of MYH9 -RD, defective myosin IIA could promote premature proPLT formation in the osteoblastic niche through loss of attenuation, or result in defective proPLT formation and reduced or abnormal PLT release in the vasculature [21] . Indeed, patients with autosomal dominant inherited MYH9 -RDs (for example, May-Hegglin anomaly) generally exhibit macrothrombocytopaenia as well as variable degrees of hearing loss, nephritis and cataracts [21] . Here we provide a mathematical model of circular-prePLT to barbell-proPLT conversion that is based on the balance of microtubule bundling forces, elastic bending forces, and actin-spectrin-myosin cortex forces. Biophysical modelling of the cytoskeletal forces driving barbell-proPLT conversion provide insight into PLT size determination that will be used to study human macrothrombocytopaenias. A better understanding of the cytoskeletal mechanisms that regulate PLT formation will lead to the development of improved therapies for clinical disorders of PLT production and an important source of PLTs for infusion. Megakaryocyte suspension cultures Mouse FLCs were collected from WT CD1 mice (Charles River Laboratories, Wilmington, MA) on day E13. 5, and cultured at 37 °C and 5% CO 2 in the presence of 0.1 μg ml −1 purified recombinant mouse c-Mpl ligand for 5 days. Round MKs, proPLT-MKs and released proPLTs were isolated by BSA gradient sedimentation, and cultured separately as previously described [7] . All studies complied with institutional guidelines approved by the Boston Children's Hospital animal care and use committee, and the IACUC. Human/murine whole-blood PLTs Human blood was obtained by venipuncture from healthy volunteers, as previously described [22] , and collected into 0.1-volume AJ buffer (85 mM sodium citrate, 69 mM citric acid, 20 mg ml −1 glucose) or Sodium Citrate (blue-capped), EDTA (purple-capped), and Heparin (green-capped) anticoagulant tubes. Collections were performed in accordance with ethics regulation with IRB approval, and informed consent was provided according to the Declaration of Helsinki. Murine blood was obtained by retro-orbital bleed into 0.1-volume AJ anticoagulant from anaesthetized CD1 strain mice, as previously described [23] . For RAMPS-treated mice, CD1 strain mice were injected with 50 μl RAMPS (Inter-cell technologies, Jupiter, FL) intraperitoneally to induce thrombocytopenia. Whole blood was collected on Day 4 post-injection, as PLT counts were recovering, and again 2 weeks later (normal control). Samples were centrifuged at 1,000 g for 5 min to isolate PRP, and stored at 37 °C and 5% CO 2 with gentle rotation for 0 or 6 h. Immunofluorescence microscopy Megakaryocytes, proPLT-MKs, released proPLTs, and whole-blood PLTs were purified and probed, as previously described [24] . Briefly, samples were fixed in 4% formaldehyde and centrifuged onto poly- L -lysine (1 μg ml −1 )-coated coverslides (resting), or spun directly onto poly- L -lysine-coated coverslides and allowed to spread for 20 min at room temperature before fixation (spread). For analysis of cytoskeletal components, samples were permeabilized with 0.5% Triton-X-100, and blocked in immunofluorescence blocking buffer (0.5 g BSA, 0.25 ml 10% sodium azide, 5 ml FCS, in 50 ml 1×PBS) overnight before antibody labelling [25] . To delineate the microtubule cytoskeleton, samples were incubated with a rabbit polyclonal primary antibody for human β1-tubulin generated against the carboxy-terminal peptide sequence CKAVLEEDEEVTEEAEMEPEDKGH (Genemed Synthesis, San Antonio, TX), washed, and probed with a secondary Alexa 488 nm-conjugated goat anti-rabbit antibody (Invitrogen). For examination of PLT surface receptor expression in non-permeabilized cells, samples were kept resting, fixed and centrifuged onto poly- L -lysine-coated coverslides as described without the 0.5% Triton-X-100 incubation, and probed with fluorescein isothiocyanate (FITC)-conjugated antibodies against GPIIIa (Beckton Dickinson). To correct for background fluorescence and nonspecific antibody labelling, slides were incubated with the secondary antibody alone or a PE-conjugated IgG antibody control, and all images were adjusted accordingly. Samples were examined with a Zeiss Axiovert 200 (Carl Zeiss, Thornwood, NY) equipped with a ×63 (NA=1.4) Plan-ApoChromat oil immersion objective, and images were obtained using a Hamamatsu charged coupled device camera (Bridgewater, NJ). Images were analysed using the Metamorph image analysis software (Molecular Devices, Sunnyvale, California, USA) and ImageJ (NIH, http://rsb.info.nih.gov/ij/ ). Blood smears Human whole-blood smears were generated by placing a 5–l drop at one end of a conventional glass slide and pulling the drop along the length of the slide using a second glass slide at a 45° angle. Blood smears were fixed and Giemsa-stained using the Diff-Quick staining kit as per the manufacturer's instructions (Siemens, Washington, DC). Laser scanning cytometry Platelet-rich plasma was spun down onto poly- L -lysine-coated glass coverslides, fixed, permeabilized, and probed for β1-tubulin, as previously described. Laser scanning cytometry was performed on the iCys Research Imaging Cytometer (CompuCyte, Westwood, Massachusetts, USA); a microscope-based cytofluorometer that employs wide-field laser-spot scanning illumination, and was used to detect β1-tubulin localization in our samples at 488 nm (ref. 26 ). Briefly, coverslides were scanned at a ×20 magnification (low-resolution mosaic scan) to generate DIC and fluorescence image maps of the sample slides. Fifty '5×5' regions of interest were selected from these image maps to uniformly represent the entire sample preparation while avoiding air-bubbles, coverslide borders, and imperfections in the glass. Samples were then scanned using a ×60 objective (field scan) to generate fluorescence region maps composed of 25 high-resolution images. These were processed using manufacturer-developed modules to threshold individual objects based on known human PLT parameters and contour these events for subsequent quantitative analysis. Data were subject to morphological and signal-level-dependent scattergram analysis using the iCys image analysis software (CompuCyte), and barbell-proPLTs, 'figure 8' proPLTs, circular-prePLTs, resting PLTs and activated PLTs were gated based on a combination of area, perimeter, circularity, integral, fluorescence intensity, and maximum pixel intensity. For the purposes of exactness in all subsequent quantifications, figure '8' proPLTs, activated PLTs, and PLT clumps were excluded from the analysis. Analysis of barbell-proPLT, circular-prePLT, and discoid PLT numbers were performed for at least three independent samples. Error bars represent 1 s.d. about the mean. Statistical significance between 0–and 6 h time points was established using a one-tailed Student's t -test for paired samples (* P <0.05, ** P <0.01). Red blood cell lysis Whole blood was collected as described above, and immediately fixed with 1% or 0.1%. formaldehyde. Samples were transferred into 2 volume equivalents of RBC lysis buffer (150 mM NH 4 Cl, 10 mM KHCO 3 , 0.1 mM EDTA, pH 7.2–7.4) and incubated at 37 °C for 10 min. PLTs were centrifuged at 1,000 g for 10 min to concentrate barbell-proPLTs/circular-prePLTs, and the resultant PLT pellet was washed briefly and then resuspended in PLT resuspension buffer (10 mM HEPES, 140 mM NaCl, 3 mM KCl, 0.5 mM MgCl 2 , 5 mM NaHCO 3 , 10 mM glucose, pH 7.4). Flow cytometry Washed PLTs/PPLTs were collected from whole blood and examined under resting conditions. Samples were probed with FITC-conjugated antibodies against CD61, and PE-conjugated antibodies against CD62P (Beckton Dickinson, Franklin Lakes, NJ) and run on a FACSCalibur flow cytometer (Beckton Dickinson). PLTs/PPLTs were gated by their characteristic forward- and side-scattering as they passed through the detector, and their total fluorescence intensity was calculated after subtraction of a FITC- or PE-conjugated IgG antibody specificity control (Beckton Dickinson). Analysis of PLT/PPLT mean fluorescence intensity was performed for at least three different samples. Error bars represent 1 s.d. about the mean for at least 3 independent samples. Electron microscopy For thin-section electron microscopy, human PLTs were fixed with 1.25% paraformaldehyde, 0.03% picric acid, 2.5% glutaraldehyde in 0.1–M cacodylate buffer (pH 7.4) for 1 h, post-fixed with 1% osmium tetroxide, dehydrated through a series of alcohols, infiltrated with propylene oxide, and embedded in epoxy resin. Ultrathin sections were stained and examined with a Tecnai G2 Spirit BioTwin electron microscope (Hillsboro, OR) at an accelerating voltage of 80 kV. Images were recorded with an Advanced Microscopy Techniques (AMT) 2-K charged coupled device camera, using AMT digital acquisition and analysis software (Advanced Microscopy Techniques, Danvers, MA). For negative stain electron microscopy, samples were fixed with 0.25% formaldehyde, lysed in 60 mM Pipes, 25 mM Hepes, 10 mM EGTA, 2 mM MgCl2 (PHEM buffer) containing 0.5% Triton X-100, and immediately centrifuged on the surface of carbon-formar-coated copper grids at 280 g . Grids were stained with 1% uranyl acetate, and viewed in a JEOL 1200 electron microscope at an accelerating voltage of 60 kV. Drug treatments Samples were incubated with 5 μM nocodazole (Sigma-Aldrich, St. Louis, Missouri, USA), 2.5 μM latrunculin, 10 μM cytochalasin D, 5 μM jasplankinolide (Invitrogen) or DMSO (vector control, Sigma-Aldrich) for up to 6 h at 37 °C. Preparation of photomicrographs The digital images produced in Metamorph were assembled into composite images by using ImageJ and Adobe Photoshop CS3 (Adobe Systems, San Jose, CA). Dividing lines explicitly separate different images, or separate regions of the same image. No specific features within an image were enhanced, obscured, moved, removed, or introduced, and adjustments made to the brightness, contrast, and colour balance were linearly applied to the whole image. How to cite this article: Thon, J. N. et al . Microtubule and cortical forces determine platelet size during vascular platelet production. Nat. Commun. 3:852 doi: 10.1038/ncomms1838 (2012).